GWAS and colocalization analyses implicate carotid intima-media thickness and carotid plaque loci in cardiovascular outcomes Carotid artery intima media thickness (cIMT) and carotid plaque are measures of subclinical atherosclerosis associated with ischemic stroke and coronary heart disease (CHD). Here, we undertake meta-analyses of genome-wide association studies (GWAS) in 71,128 individuals for cIMT, and 48,434 individuals for carotid plaque traits. We identify eight novel susceptibility loci for cIMT, one independent association at the previously-identified PINX1 locus, and one novel locus for carotid plaque. Colocalization analysis with nearby vascular expression quantitative loci (cis-eQTLs) derived from arterial wall and metabolic tissues obtained from patients with CHD identifies candidate genes at two potentially additional loci, ADAMTS9 and LOXL4 . LD score regression reveals significant genetic correlations between cIMT and plaque traits, and both cIMT and plaque with CHD, any stroke subtype and ischemic stroke. Our study provides insights into genes and tissue-specific regulatory mechanisms linking atherosclerosis both to its functional genomic origins and its clinical consequences in humans. Atherosclerosis is characterized by an accumulation of lipid-rich and inflammatory deposits (plaques) in the sub-intimal space of medium and large arteries. Plaque enlargement leads to blood flow limitation, organ ischemia, and/or tissue necrosis. Plaque rupture can lead to abrupt vascular occlusion, which underlies clinical cardiovascular events, including myocardial infarction and ischemic stroke. Coronary heart disease (CHD) accounts for one in seven deaths, and stroke accounts for one in 20 deaths in the US [1] . Because atherosclerosis has a long pre-clinical phase, early detection of atherosclerosis using non-invasive methods may help identify individuals at risk for atherosclerotic clinical events [2] , and provides an opportunity for prevention. Subclinical atherosclerosis can be detected by B-mode ultrasound measurement of common carotid artery intima-media thickness (cIMT) or carotid plaques [1] . Subclinical and clinical atherosclerosis has known genetic components [3] . Genome-wide association studies (GWAS) of subclinical atherosclerosis have previously identified three loci significantly associated with cIMT at ZHX2 , APOC1 , and PINX1 , and two loci associated with common carotid artery plaque at PIK3CG and EDNRA [4] . An exome-wide-association study identified significant associations of the APOE ε2 allele with cIMT and coronary artery calcification [5] . The APOE single nucleotide polymorphism (SNP) rs7412 is in linkage disequilibrium (LD) with the APOC1 variant, thus representing the same signal. Additional GWAS-identified associations were reported for carotid plaque at the 9p21 and SFXN2 loci [6] , and for cIMT at the CFDP1 - TMEM170A locus [7] . However, these prior studies were of limited sample size and genomic coverage, and failed to investigate the etiological role that subclinical atherosclerosis may have on atherosclerotic clinical events. Herein, we perform a large meta-analysis of GWAS of subclinical atherosclerosis by analyzing 1000 Genomes imputed genotype data obtained from collaborations between the Cohorts for Heart and Aging Research in Genomic Epidemiology (CHARGE) consortium [8] and the University College London-Edinburgh-Bristol (UCLEB) consortium [9] . One of the greatest challenges in the translation of GWAS findings to biological understanding is related to the limited access to RNA expression data from disease-relevant tissues. Consequently, we sought to reliably identify the tissue-specific gene regulatory functions responsible for the GWAS signals by prioritizing candidate genes for established and novel loci of cIMT and carotid plaque using statistical methods for colocalization [10] . These methods integrate identified loci with expression quantitative loci (eQTLs) inferred from cardiovascular disease-relevant genetics of RNA expression, the Stockholm-Tartu Atherosclerosis Reverse Network Engineering Task (STARNET) study, where arterial wall and metabolic-related RNA samples were collected from up to 600 patients with CHD [11] . We also evaluate the relationships of cIMT and carotid plaque with clinically apparent CHD and stroke using summary data from two large consortia. In summary, our study sequentially assesses the genetic epidemiology and tissue-specific patterns of gene regulation involved in the formation of subclinical atherosclerosis traits across cardiovascular disease-related tissues. Study description The study design is shown in Fig. 1 . 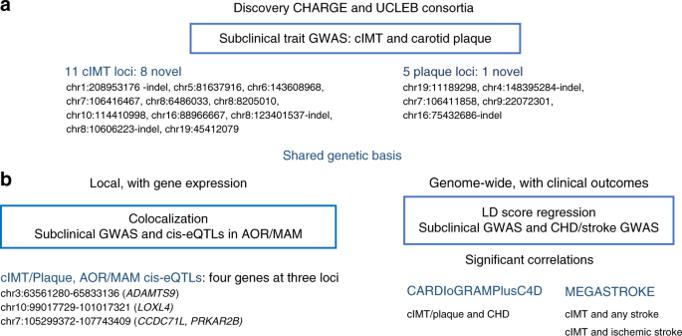Fig. 1 Overall study design.aGWAS meta-analyses of cIMT and carotid plaque for gene discovery.bLocal and genome-wide shared genetic basis using gene expression and clinical outcomes GWAS data We undertook meta-analysis of GWAS in individuals of European ancestry for cIMT (up to 71,128 participants from 31 studies) and carotid plaque (up to 48,434 participants from 17 studies; 21,540 with defined carotid plaque) (Supplementary Table 1 ). cIMT and plaque were evaluated using high-resolution B-mode ultrasonography and reading protocols as previously reported [4] . 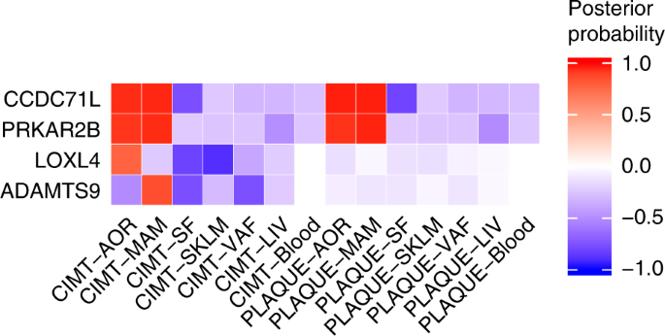Fig. 2 Pairwise colocalization results for genes identified for cIMT and carotid plaque GWAS meta-analysis with STARNET expression datasets. Red indicates a high posterior probability of colocalization and blue a high probability of no colocalization of the same SNP with tissue eQTLs Carotid plaque was defined by atherosclerotic thickening of the common carotid artery wall or the proxy measure of luminal stenosis greater than 25% (Supplementary Table 2 ). Each cohort performed association analyses using standardized protocols (Methods) for variants imputed based on the 1000 Genomes Project (1000G) phase 1 v3 reference. 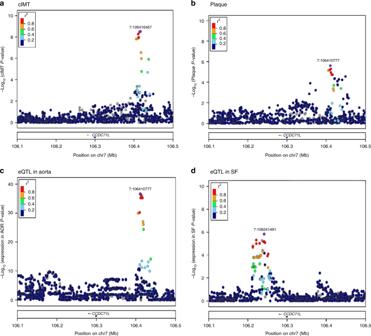Fig. 3 Association results at theCCDC71Llocus (chromosome 7), showing a high posterior probability of a shared variant for cIMT and carotid plaque in AOR and MAM eQTLs. −log10(p) SNP associationp-values for cIMT (plot A) and carotid plaque (plot B), and eQTL in AOR (plot C) and eQTL in SF (plot D). Association results in SF tissue have a low probability of a shared signal with cIMT and carotid plaque, possibly indicating a different mechanism in this tissue. eQTLs in MAM are identical to AOR and not shown. Thep-values were calculated by fitting a linear regression model with cIMT or plaque as dependent variable and imputed SNPs as independent variables. Each dot is an SNP and the color indicates linkage disequilibrium (r2) with the best hit (in purple) Extensive quality control (QC) was applied to data, and there was little evidence for population stratification in any of the studies for either trait (Supplementary Table 3 ). The study-specific results were combined using fixed-effect meta-analyses, given the low heterogeneity across studies (0% heterogeneity) [12] . Fig. 1 Overall study design. a GWAS meta-analyses of cIMT and carotid plaque for gene discovery. b Local and genome-wide shared genetic basis using gene expression and clinical outcomes GWAS data Full size image GWAS meta-analyses of cIMT and carotid plaque For cIMT, 11 loci had at least one SNP association that reached the genome-wide association threshold ( p < 5 × 10 −8 ), of which eight were newly described and three have been previously reported (Table 1 ). The closest genes for the eight loci were: 1q32.2 intergenic (rs201648240), ATP6AP1L (rs224904), AIG1 (rs6907215), PIK3CG (rs13225723), MCPH1 (rs2912063), SGK223 (rs11785239), VTI1 (rs1196033), and CBFA2T3 (rs844396). For three loci previously reported, the closest genes were ZHX2 (rs148147734), PINX1 (rs200482500), and APOE (rs7412). Table 1 Loci significantly associated with cIMT and plaque GWAS Full size table The PIK3CG is a newly described locus for cIMT, but has been previously reported in a GWAS of carotid plaque [4] . The two signals on chromosome 8 near MCPH1 (rs2912063) and SGK223 (rs11785239) were confirmed to be independent through conditional analysis (Supplementary Table 4 ). At the PINX1 locus, the lowest association p -value variant (rs200482500) was not in LD with the previously reported associated variant in the region (rs6601530, r 2 = 0.0, Table 1 ), thus representing an independent signal at this locus. Two additional loci for cIMT had an SNP that reached suggestive evidence for association ( p < 1.0 × 10 −7 ) including an SNP nearby APOB (rs515135) and an intronic low frequency variant at ATG4B (rs139302128, minor allele frequency [MAF] = 0.03) (Supplementary Table 5 ). The GWAS meta-analysis for carotid plaque identified five loci, of which one has not been previously described (nearby gene LDLR ) (Table 1 ). At four known loci associated with carotid plaque (nearby genes EDNRA , PIK3CG , CFDP1-TMEM170A , and at the 9p21 region), the most significantly associated variants were in LD with the previously reported SNPs (Table 1 ) [4] , [6] , [7] , indicating that these SNPs mark the same association at each locus. Two suggestive loci ( p < 10 −7 ) were also identified nearby the genes TMCO5B and STEAP2-AS1 (Supplementary Table 5 ). Conditional analyses confirmed the presence of a single independent signal at each locus. Manhattan and QQ plots from the meta-analysis of cIMT and carotid plaque are shown in Supplementary Figure 1 and regional plots in Supplementary Figure 2 . Forest Plots for all loci are shown in Supplementary Figure 3 . Regulatory annotations of GWAS SNPs for cIMT/carotid plaque To better define potentially causal variants within the identified genetic risk loci, we jointly analyzed the GWAS data with functional genomic information such as annotations on active transcription sites or open chromatin regions (i.e., performed a fine-mapping functional genome-wide association analysis using fGWAS [13] ). Only variants in the PINX1 region were found to have a high probability that its association with cIMT is driven by SNPs that fall within transcription sites in adipose-derived mesenchymal stem cells at a DNaseI-hypersensitive site (Supplementary Figure 4 ), a finding that provides a down-stream mechanistic explanation for the cIMT signal in the PINX1 locus. To further explore the regulatory functions of variants in the identified loci for cIMT and carotid plaque, we investigated whether the identified lead SNPs were also eQTLs using vascular RNAseq data from GTEx (aorta, coronary and tibial arteries, heart atrial appendage, and heart left ventricle) and from the coronary artery disease cohort of STARNET (i.e., from the atherosclerotic-lesion-free internal mammary artery [MAM] and atherosclerotic aortic root [AOR]). Lead SNP associated with cIMT and carotid plaque (rs13225723) in the PIK3CG locus was found to be vascular-specific eQTLs for CCDC71L and PRKAR2B in GTEx aorta as well as in STARNET AOR and MAM tissues (Table 2 , Fig. 2 ), suggesting that the genetic regulation of these two genes are responsible for risk variation in cIMT and carotid plaque development in this locus. Table 2 Gene expression results for significant SNPs in GTEx and STARNET tissues Full size table Fig. 2 Pairwise colocalization results for genes identified for cIMT and carotid plaque GWAS meta-analysis with STARNET expression datasets. Red indicates a high posterior probability of colocalization and blue a high probability of no colocalization of the same SNP with tissue eQTLs Full size image Colocalization analysis of GWAS data and STARNET eQTLs To identify further candidate genes in tissues affected by atherosclerosis that had strong evidence of sharing the same variant for cIMT and carotid plaque as found in our GWAS, we conducted pairwise colocalization analysis of these genetic variants with cis -eQTLs in the STARNET study [10] . The pairwise colocalization analysis is based on coloc, a Bayesian statistical methodology that tests pairwise colocalization of SNPs in GWAS with eQTLs and, in this fashion, generates posterior probabilities for each locus weighting the evidence for competing hypothesis of either no colocalization or sharing of a distinct SNP at each locus [10] . We used summary statistics from all SNPs within a 200-kb window around each gene covered by the eQTL datasets ( N = 18,705, see Methods), and analyzed each eQTL-GWAS dataset pair (Supplementary Table 6 ). A posterior probability of ≥75% was considered strong evidence of the tissue-specific eQTL-GWAS pair influencing both the expression and GWAS trait at a particular region. Results for this analysis are shown in Table 3 and Supplementary Figure 5 . The strongest evidence for an effect on gene expression within the regions identified in our standard GWAS meta-analysis was for the CCDC71L and PRKAR2B genes at the previously described chromosome 7 cIMT locus ( PIK3CG in Table 2 , Fig. 2 ). These genes showed evidence of colocalization for both cIMT and carotid plaque in AOR and MAM tissues (Table 3 , Fig. 3 ). CCDC71L had the highest probability (>95%) for colocalization for cIMT, and MAM and AOR tissue eQTLs, and for carotid plaque, and MAM and AOR tissue eQTLs. We found a low probability of colocalization of the SNP with the PIK3CG gene expression (<1%). Table 3 Colocalization of cIMT and plaque with eQTLs in tissues from patients with CHD in STARNET tissues for genes/tissues combinations that have more than 75% probability to share the same associated variant Full size table Fig. 3 Association results at the CCDC71L locus (chromosome 7), showing a high posterior probability of a shared variant for cIMT and carotid plaque in AOR and MAM eQTLs. −log10( p ) SNP association p -values for cIMT (plot A) and carotid plaque (plot B), and eQTL in AOR (plot C) and eQTL in SF (plot D). Association results in SF tissue have a low probability of a shared signal with cIMT and carotid plaque, possibly indicating a different mechanism in this tissue. eQTLs in MAM are identical to AOR and not shown. The p -values were calculated by fitting a linear regression model with cIMT or plaque as dependent variable and imputed SNPs as independent variables. Each dot is an SNP and the color indicates linkage disequilibrium ( r 2 ) with the best hit (in purple) Full size image The eQTL associations at two additional loci ( ADAMTS9 , LOXL4 ) in MAM or AOR showed evidence of colocalization with cIMT or carotid plaque, although GWAS association p -values at these loci did not meet the genome-wide significance threshold (Table 3 , Supplementary Figure 5 ). Albeit with weaker magnitudes, the expression of these two genes were also associated with the top colocalizing SNPs as detected in RNAseq data in GTEx aorta (rs17676309, chr3:64730121, ADAMTS9 , p = 0.0003 and rs55917128, chr10:100023359, LOXL4 , p = 0.0005). Colocalization of CHD and stroke GWAS and STARNET eQTLs We next assessed if the four genes ( CCDC71L, PRKAR2B, ADAMTS9, LOXL4) identified through colocalization of cIMT/carotid plaque with tissue-specific eQTLs also showed evidence for colocalization with CHD and stroke traits (Supplementary Data 1 and Supplementary Figure 6 ). We used GWAS summary data for CHD (CARDIoGRAMPlusC4D), and stroke subtypes (MEGASTROKE) and AOR and MAM STARNET tissue eQTLs for these analyses. CCDC71L and PRKAR2B had suggestive evidence of sharing the same variant with large vessel disease stroke in both AOR and MAM tissues (probability of colocalization ≥20%, Supplementary Data 1 ). In contrast, there was strong evidence (≥75%) to reject a shared variant for CHD and eQTLs at this locus, thus suggesting there is atherosclerotic outcome specificity at vascular level for this locus (Supplementary Figure 5 ). Three of these genes, CCDC71L , PRKAR2B , and ADAMTS9 , showed evidence for shared genetic influences of cIMT or carotid plaque on CHD/stroke outcomes when testing the joint association using moloc, a multiple-trait extension of coloc [14] (Supplementary Table 7 ). We also highlight the expression of KIAA1462 gene in MAM, carotid plaque/cIMT, and CHD, which were positively correlated (Supplementary Figure 7 ). This gene has suggestive evidence of pairwise colocalization with carotid plaque (67% of probability of shared variant between carotid plaque and eQTL in MAM), as well as a high probability of shared variant between MAM eQTL expression of this gene, GWAS carotid plaque or cIMT, and CHD traits (Supplementary Table 7 ). We note, however, that the GWAS signal for outcomes across the datasets did not reach genome-wide significance and larger sample sizes may be needed to strengthen the evidence for involvement in disease outcomes. Genetic correlations of cIMT/carotid plaque and clinical outcomes To provide etiological insights into the role of measures of subclinical atherosclerosis and major atherosclerotic disease outcomes such as CHD and ischemic stroke, we quantified the genetic correlation using cross-trait LD score regression, a method that estimates genetic correlation across different traits using summary level data [15] . We used summary statistics between cIMT/carotid plaque with CHD and stroke meta-analysis of GWAS. Both cIMT and carotid plaque had positive significant genetic correlations with CHD (all p < 0.05 after adjusting for multiple testing), though the magnitude of the correlation was twice as strong for carotid plaque (0.52) as for cIMT (0.20) (Table 4 ). There was also evidence for genetic correlations between cIMT with any stroke and ischemic stroke subtype. Table 4 Genetic correlation between CHD and stroke traits with cIMT and plaque, and cIMT with plaque using LD score and meta-GWAS Full size table Pathway analysis and druggability Gene Ontology (GO) analyses of genes identified in the loci for cIMT and carotid plaque according to our meta-analysis of GWAS (Table 1 and Supplementary Table 5 ) and in the colocalization analyses (Table 3 , Supplementary Table 7 ) showed that cIMT genes are enriched in lipoprotein-related terms and cholesterol efflux, whereas carotid plaque genes are enriched in terms associated with fibroblast apoptosis (Supplementary Figure 8 ). Analysis of the cIMT genes using a GO Slim additionally identified several of the genes that were associated with terms describing cardiovascular development, cell adhesion, and immune processes, processes already considered relevant to atherosclerosis. Specifically, there is corroborating evidence from GO that CCDC71L, PRKAR2B, and TWIST1 are associated with cIMT/carotid plaque as they are involved in lipid metabolism, with similar support that ADAMTS9, CDH13, and KIAA1462 are associated with cIMT or carotid plaque risk as they are all involved in cell adhesion and, together with TWIST1 , in cardiovascular system development (Supplementary Data 2 ). From the loci associated with cIMT and carotid plaque, we identified seven genes ( ATG4B, ALPL, LDLR, APOB, EDNRA, APOE , and ADAMTS9 ) whose encoded proteins are targets at various stages of the drug development process (Supplementary Tables 8 and 9 ). ADAMTS9 gene encodes a protein likely to be druggable [16] . ATG4B, ALPL, and LDLR are proteins being targeted by compounds in pre-clinical phase (tier 2), while APOB and EDNRA are proteins targeted by drugs in clinical phase or licensed (tier 1). APOB is the target of an approved FDA drug for treatment of familial hypercholesterolemia. EDNRA gene encodes for endothelin A receptor, against which several antagonists have been developed for the treatment of pulmonary arterial hypertension or which are in advanced clinical phase development for non-small cell lung cancer and diabetic nephropathy. We provide results of a large meta-analysis of GWAS of subclinical atherosclerosis and we integrate our results with tissue-specific gene expression data using eQTLs from both the early (MAM) and late advanced (AOR) atherosclerotic arterial wall from the STARNET study to enable reliable discovery of genes with biological evidence of an increased probability for conferring inherited risk of atherosclerosis development. Our discovery approach using GWAS meta-analyses identified 16 loci significantly associated with either cIMT or carotid plaque, of which nine are novel. The integration of GWAS and tissue-specific cis -eQTLs for the joint analyses of tissue-specific eQTLs from CHD patients identified two potentially additional loci colocalizing with cIMT or carotid plaque: chr3:63561280-65833136 ( ADAMTS9 ), chr10:99017729-101017321 ( LOXL4). ADAMTS9 is a metalloproteinase involved in thrombosis and angiogenesis and has been associated with cardiometabolic traits (waist-to-hip ratio, waist circumference, and type 2 diabetes) in GWAS, and with coronary artery calcification in a gene-by-smoking interaction GWAS [17] , [18] . LOXL4 encodes a lysyl oxidase involved in crosslinks of collagen and elastin in the extracellular matrix. This family of proteins are involved in the development of elastic vessels and mechanical strength of the vessel wall, and their inhibition was associated with the development of abdominal aortic aneurysms and more severe atherosclerosis in experimental models [19] . Some loci identified in our meta-analysis of GWAS include genes in known pathways for atherosclerosis, including LDLR , which is related to lipid pathways and CHD, and identified for associations with carotid plaque in our study. For most of the loci, however, the underlying gene implicated in signals are unknown. Our colocalization approach found both CCDC71L and PRKAR2B as the most likely genes at the chromosome 7 locus, where PIK3CG was previously the suggested gene. This finding is in agreement with a targeted sequencing study of subclinical atherosclerosis [15] . An additional SNP (rs342286) at this locus has been associated with platelets volume and reactivity, and cardiovascular traits. However, rs342286 is not in LD with our most significant SNP and it is not associated with cIMT or carotid plaque in our studies ( p = 0.49 and 0.01, respectively). Of interest, the variant we identified in this study showed evidence for colocalization with cIMT/carotid plaque and large vessel disease stroke but not CHD, therefore showing tissue and outcome-specificity. CCDC71L has unknown function. PRKAR2B codes for one of the several regulatory subunits of cAMP-dependent protein kinase and its expression is ubiquitous. In vitro studies have shown that adenosine-induced apoptosis of arterial smooth muscle cells involves a cAMP-dependent pathway [20] . Measures of cIMT and carotid plaque reflect vascular pathophysiologic and atherosclerosis processes, respectively, with carotid plaque more strongly reflecting atherosclerotic clinical events. An important contribution of this study is the supporting evidence for overall genetic correlations of CHD and stroke (any cause and ischemic stroke) with subclinical atherosclerosis traits, estimated using LD score methods. Further highlighting the potential biological relevance of our findings, the genetic correlations estimates for CHD were stronger for carotid plaque than for cIMT. However, cIMT and carotid plaque GWAS were correlated, and the genetic correlations estimates with stroke were similar for cIMT or carotid plaque, and not significant for carotid plaque. The colocalization analyses provided additional insights in the relationships between subclinical atherosclerosis, clinical outcomes, and tissue-specific regulation at specific genomic regions. For example, our suggestive top gene association in multi-trait colocalization for KIAA1462 included MAM eQTLs, carotid plaque, and CHD, supporting the shared genetic effects at this locus of atherosclerosis in carotid and coronary arteries. KIAA1462 has been previously reported in the same locus identified by GWAS for CHD [21] . This gene encodes a protein involved in cell–cell junctions in endothelial cells [22] , which was recently shown to be involved in pathologic angiogenic process in in vitro and in vivo experimental models [23] . These findings suggest that there may be important differences in vascular bed regulation at distinctive regions for atherosclerotic cardiovascular and stroke outcomes that may help to identify genes and specific targets for CHD or stroke prevention and treatment. Additional studies in diverse and large samples across the multiple datasets are needed to explore these results further. As more summary statistics become available for other clinical end-points beyond stroke and CHD (both in terms of larger sample size and richer genome coverage), and as further refinements in clinical phenotypes emerge (e.g. from CHD to acute coronary syndrome sub-components), strategies to integrate this knowledge using methods such as moloc [10] and eCAVIAR [24] will continue to be essential for harnessing genome-wide findings in the drug-discovery process. In summary, our study is a large GWAS meta-analysis of cIMT and carotid plaque. Through a sequential approach of discovery and colocalization studies, we provide deeper insights into disease causal genes of subclinical cIMT and carotid plaque formation. We confirmed three loci and identified nine novel loci in the meta-analyses of cIMT and carotid plaque. Additionally, we provide strong evidence for the role of three novel genes from our integrative analysis of GWAS and eQTL data. Moreover, the identified correlations with CHD and stroke highlight novel biological pathways that merit further assessments as novel targets for drug development. Ethics statement All human research was approved by the relevant institutional review boards for each study, and conducted according to the Declaration of Helsinki. All participants provided written informed consent. Populations and phenotypes The discovery GWAS in this study consists of a collaboration between the CHARGE [8] and the UCLEB consortia [9] , for genetic studies of cIMT and carotid plaque among individuals of European ancestry (Supplementary Note 1 ). All studies followed standardized protocols for phenotype ascertainment and statistical analyses. The descriptive characteristics of participating studies are shown in Supplementary Table 1 . cIMT and carotid plaque measures were evaluated using high-resolution B-mode ultrasonography and reading protocols as previously reported [4] . We used data from the baseline examination or the first examination in which carotid ultrasonography was obtained. cIMT was defined by the mean of the maximum of several common carotid artery measurements, measured at the far wall or the near wall. For most studies, this was an average of multiple measurements from both the left and right arteries. We also examined a carotid plaque phenotype, defined by atherosclerotic thickening of the carotid artery wall or the proxy measure of luminal stenosis greater than 25% (Supplementary Table 2 ). Genotyping, imputation, and study-level quality control Genotyping arrays and QC pre-imputation are shown in Supplementary Table 3 . Each GWAS study conducted genome-wide imputation using a Phase 1 integrated (March 2012 release) reference panel from the 1000G Consortium using IMPUTE2 [25] or MaCH/minimac [26] , and used Human Reference Genome Build 37. Sample QC was performed with exclusions based on call rates, extreme heterozygosity, sex discordance, cryptic relatedness, and outlying ethnicity. SNP QC excluded variants based on call rates across samples and extreme deviation from Hardy–Weinberg equilibrium (Supplementary Table 3 ). Non-autosomal SNPs were excluded from imputation and association analysis. Pre-meta-analysis GWAS study-level QC was performed using EasyQC software [27] . This QC excluded markers absent in the 1000G reference panel; non A/C/G/T/D/I markers; duplicate markers with low call rate; monomorphic SNPs and those with missing values in alleles, allele frequency, and beta estimates; SNPs with large effect estimates or standard error (SE) ≥10; and SNPs with allele frequency difference >0.3 compared to 1000G reference panel. There was a total of 9,574,088 SNPs for the cIMT meta-analysis and 8,578,107 SNPs for the carotid plaque meta-analysis. Statistical analyses Within each study, we used linear and logistic regression to model cIMT and carotid plaque, respectively, and an additive genetic model (SNP dosage) adjusted for age, sex, and up to 10 principal components. We combined summary estimates from each study and each trait using an inverse variance weighted meta-analysis. Additional filters were applied during meta-analyses including imputation quality (MACH r 2 < 0.3 and IMPUTE info <0.4), a minor allele frequency (MAF) <0.01, and SNPs that were not present in at least four studies. The genome-wide significance threshold was considered at p < 5.0 × 10 −8 . To assess the evidence for independent associations at each locus attaining genome-wide significance, we performed conditional analysis in a 1-Mb genomic interval flanking the lead SNP using GCTA [28] . This approach uses summary meta-analysis statistics and a LD matrix from an ancestry-matched sample to perform approximate conditional SNP association analysis. The estimated LD matrix was based on 9713 unrelated individuals of European ancestry from the ARIC study, which was genotyped using an Affymetrix 6.0 array and imputed to the 1000G panel using IMPUTE2 [25] . Gene expression analysis using GTEx GTEx Analysis V6 (dbGaP Accession phs000424.v6.p1) eQTL results were downloaded from GTEx portal for 44 tissues, and then mapped to SNPs listed in Table 1 . We used a false discovery rate (FDR) of ≤0.05. Colocalization analyses using eQTLs We integrated our GWAS results with cis- eQTL data using a Bayesian method (coloc) [10] . This method evaluates whether the GWAS and eQTL associations best fit a model in which the associations are due to a single shared variant (summarized by the posterior probability). We used gene expression datasets from multiple tissues from patients with CHD of the STARNET study, including blood, MAM, AOR, subcutaneous fat (SF), visceral fat (VAF), skeletal muscle (SKLM), and liver (LIV) obtained from 600 patients during open heart surgery [11] . Pairwise colocalization was tested between these expression disease tissue datasets and GWAS results from our cIMT/carotid plaque GWAS meta-analysis. We used GWAS and eQTL summary statistics of SNPs within a 200-kb window around each gene covered by the eQTL datasets. A posterior probability of colocalization ≥0.75 was considered a strong evidence for a causal gene. Next, we reported the gene(s) in the STARNET datasets that had the strongest evidence of sharing the same variant with cIMT or carotid plaque genome-wide. In an alternative analysis, we also tested loci with an SNP that reached a threshold of significant or suggestive genome-wide significance for cIMT or carotid plaque (reported in Table 1 , Supplementary Table 5 ). For each region 200kb around the SNP with the lowest association p -value, we report the gene with the highest probability of being responsible for the GWAS signal (Supplementary Table 6 ). Pairwise colocalization for these genes was also tested for publicly available GWAS for CHD case-controls (CARDIoGRAMPlusC4D) and stroke case-controls (MEGASTROKE consortium). The MEGASTROKE dataset uses genotypes imputed to the 1000G phase I haplotype panel. The European ancestry sample used to generate these results consisted of 40,585 stroke cases and 406,111 controls from 15 cohorts and two consortia: the METASTROKE and CHARGE consortia [29] . The phenotypes used in this analysis were any stroke ( n = 39,067 cases, total n = 442,142), ischemic stroke (IS, n = 32,686 cases, total n = 423,266), and etiologic stroke subtypes:cardioembolic stroke (CE, n = 6,820 cases, total n = 314,368), large vessel disease ( n = 4,113, total n = 202,263), and small vessel disease (SVD, n = 4,975, total n = 242,250). To explore multi-trait colocalizations, we used moloc [14] with prior probabilities of 10 −4 for GWAS/GWAS/eQTL, 10 −6 for GWAS+eQTL/GWAS or GWAS+GWAS/eQTL, and 10 −7 for colocalization of all three association signals. Functional annotation and epigenetic enrichment analyses From the Epigenome Roadmap Project [30] , [31] , we obtained regulatory information using broad classes of chromatin states ( n = 127 tissues) capturing promoter-associated, transcription-associated, active intergenic, and large-scale repressed and repeat-associated states. From ENCODE [32] , we obtained chromatin states, uniformly processed transcription factor (TF) Chip assays and DNaseI Hypersensitivity sites (DHS) for nine cells lines. From FANTOM5 [33] , we used information from expression of enhancers in each tissue ( n = 112), and enhancers that are positively differentially expressed against any other tissue ( n = 110). We used fGWAS [13] to identify genomic annotations that are enriched within the cIMT results and to select the variants with support for a functional role based on the most informative annotations. We only considered cIMT for these analyses because of the small number of identified loci for carotid plaque. We first estimated the enrichment parameters for each annotation individually and identified the set of annotations with significant marginal associations. We then applied 10-fold cross-validation likelihood and forward selection to identify the set of annotations that significantly improve the model fit, and reverse selection of each annotation included in the model, as suggested in the fGWAS workflow. We reported the model with the highest cross-validation likelihood and SNPs that have regional posterior probability of association (PPA) >0.9 and directly overlap the genomic annotations considered. Overall genetic correlation analysis Genetic correlation between cIMT/carotid plaque, CHD, and stroke traits were calculated using LD score regression approach LD-score, which uses GWAS summary statistics and is not affected by sample overlap. This method relies on the fact that the χ 2 association statistic for a given SNP includes the effects of all SNPs that are in LD with it and it calculates genetic correlation by partitioning the SNP heritabilities [15] . Genetic correlations between stroke traits (IS, CE, large vessel disease, and SVD) and cIMT and carotid plaque were calculated using software available at http://github.com/bulik/ldsc with GWAS summary statistics for our cIMT/carotid plaque GWAS, CARDIOGRAMPlusC4D data, and stroke GWAS. We used the LD-scores [15] , which are based on the 1000 Genomes European population and estimated within 1-cM windows. Based on ten tests performed (two subclinical traits and five outcomes), we set the significance threshold to p = 0.005. PATHWAY ANALYSES . Methods for GO Slim : The Ensembl identifiers of all protein-coding genes identified as in LD with the 12 variants for cIMT and 15 variants for carotid plaque (including variants from main and suggestive signals, Table 1 and Supplementary Table 5 ), and five genes for which there is strong evidence of colocalization (Table 3 ), were mapped to UniProt accession numbers, using the UniProt ID mapping service ( http://www.uniprot.org/uploadlists/ ). A GO Slim analysis was performed on this list using QuickGO (www.ebi.ac.uk/QuickGO) and the Generic GO Slim. The GO terms used in the final slim analysis were further refined by adding/removing GO terms to provide more detailed information about the processes covered. Methods for GO term enrichment analysis : The VLAD gene list analysis and visualization tool ( http://proto.informatics.jax.org/prototypes/vlad/ ) was used to perform a GO term enrichment analysis on the same UniProt accessions as listed for the GO Slim. The background annotation set was obtained from the goa_human.gaf file (dated 21 November 2017, downloaded from ftp://ftp.ebi.ac.uk/pub/databases/GO/goa/HUMAN/) and the ontology data was obtained from the go-basic.obo file provided in the VLAD tool (analysis run 28 November 2017). The LD block around top SNPs associated with cIMT and carotid plaque was constructed using LD information from the 1000 Genomes panel, as previously outlined in Finan et al. [16] . Briefly, the boundaries of the LD region were defined as the positions of the variants furthest upstream and downstream of a GWAS SNP with an r 2 value of ≥0.5 and within a 1-Mbp flank on either side of the GWAS variant. Associated variants that were not present in the 1000 Genomes panel that were not in LD with any other variants were given a nominal flank of 2.5 kbp on either side of the association. Gene annotations using Ensembl version 79 were then overlapped to the LD region. Druggable genes We examined the druggability status for the nearest coding genes identified in our GWAS analysis on cIMT and carotid plaque, including significant (novel and replicated) and suggestive ones, as well as genes identified through colocalization analysis. The druggable gene set was calculated using the previously described criteria: novel targets of first-in-class drugs licensed since 2005; the targets of drugs currently in late phase clinical development; pre-clinical phase small molecules with protein binding measurements reported in the ChEMBL database; and genes encoding secreted or plasma membrane proteins that are targets of monoclonal antibodies and other bio-therapeutics [16] . We defined three tiers of druggable gene sets based on their drug development. In Tier 1, 1427 genes were targets of approved small molecules and biotherapeutic drugs and clinical-phase drug candidates. Tier 2 comprised 682 genes encoding targets with known bioactive drug-like small molecule binding partners and those with significant sequence similarity to approved drug targets. Tier 3 contained 2370 genes encoding secreted or extracellular proteins, proteins with more distant similarity to approved drug targets, and druggable genes not included in Tier 1 or 2 such as GPCRs, nuclear hormone receptors, ion channels, kinases, and phosphodiesterases. URLs For GTEx, see http://gtexportal.org/ . For Coloc, see https://cran.r-project.org/web/packages/coloc/coloc.pdf . For, Moloc, see https://github.com/clagiamba/moloc/blob/master/man/moloc-package.Rd . For CARDIoGRAMPlusC4D, see www.cardiogramplusc4d.org/ . For LD scores, www.broadinstitute.org/~bulik/eur_ldscores/ . For UniProt ID, www.uniprot.org/uploadlists/ . For QuickGO, www.ebi.ac.uk/QuickGO . For VLAD tool, see http://proto.informatics.jax.org/prototypes/vlad/ .